An assay to image neuronal microtubule dynamics in mice Microtubule dynamics in neurons play critical roles in physiology, injury and disease and determine microtubule orientation, the cell biological correlate of neurite polarization. Several microtubule binding proteins, including end-binding protein 3 (EB3), specifically bind to the growing plus tip of microtubules. In the past, fluorescently tagged end-binding proteins have revealed microtubule dynamics in vitro and in non-mammalian model organisms. Here, we devise an imaging assay based on transgenic mice expressing yellow fluorescent protein-tagged EB3 to study microtubules in intact mammalian neurites. Our approach allows measurement of microtubule dynamics in vivo and ex vivo in peripheral nervous system and central nervous system neurites under physiological conditions and after exposure to microtubule-modifying drugs. We find an increase in dynamic microtubules after injury and in neurodegenerative disease states, before axons show morphological indications of degeneration or regrowth. Thus increased microtubule dynamics might serve as a general indicator of neurite remodelling in health and disease. The microtubule cytoskeleton plays a critical role in the establishment and maintenance of neuronal polarization [1] and is crucial for intracellular transport in axons and dendrites. Contrary to what the term ‘skeleton’ implies, microtubules are highly dynamic structures constantly being assembled and disassembled [2] . The maintenance of microtubule structure and orientation is hence an important aspect of neuronal homeostasis with loss of microtubules often representing an early stage of neurite dismantling—both during normal development [3] , [4] and under pathological conditions [5] , [6] , [7] . Microtubule dynamics can be assayed using fluorescently tagged end-binding proteins (EBs) [8] , [9] , a technique that has thus far been applied in vitro and in non-mammalian model systems [10] , [11] , [12] , [13] . EB imaging has proven to be an efficient and non-toxic approach to reveal the density and orientation of dynamic microtubules. However, investigating the role of microtubule dynamics in mature mammalian neurons has, to our knowledge, not been possible yet. To assay such dynamics by in vivo imaging in the mammalian nervous system, we generated transgenic mice that express EB3 fused to yellow fluorescent protein (YFP) controlled by neuron-specific Thy1 promoter elements, which have been used previously to generate numerous versatile reporter mice of neuronal morphology, function and organelles [14] , [15] , [16] , [17] . When matched by appropriate forms of in vivo microscopy, our approach now allows quantifying microtubule dynamics in a wide range of central and peripheral neurites under physiological conditions, after injury and during chronic neurodegeneration. Characterization of Thy1:EB3-YFP transgenic mice The three Thy1 :EB3-YFP transgenic lines (J045, J023, J030) that we characterized in detail showed YFP fluorescence in a broad spectrum of neurons in the central nervous system (CNS) and peripheral nervous system (PNS), but varied in brightness and percentage of expressing cells ( Supplementary Fig. 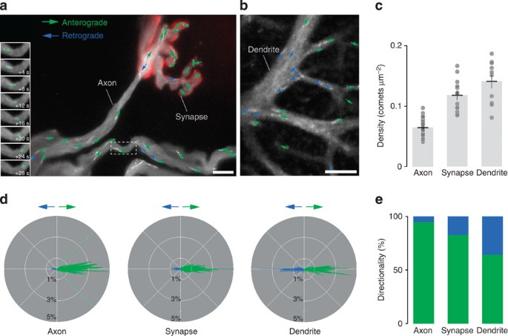Figure 1: Imaging microtubule dynamics inThy1:EB3-YFP mice. (a) A neuromuscular junction (postsynaptic receptors labelled with fluorescently tagged Bungarotoxin, red) and terminal motor axons in an acuteThy1:EB3-YFP triangularis sterni explant. Inset shows eight frames cropped (dashed box in main panel) from a time-lapse sequence of this area highlighting an anterogradely directed EB3 comet (pseudocolored in green). The main panel shows a maximum intensity projection of 20 s within the time lapse (for full movie, seeSupplementary Movie 1online), where each comet is represented by a colour-coded arrow (anterograde, green; retrograde, blue). (b) Dendrite of a Purkinje cell in an acute cerebellar slice represented in the same way as in (a) (seeSupplementary Movie 3). Note the more frequent occurrence of retrogradely directed comets. (c) Comet density in different neuronal compartments (n≥10 neurites from ≥3 mice for each group; horizontal line shows mean±s.e.m.). (d) Polar plots (that is frequency histograms with angular orientation shown in a circle) of comet directionality in relation to neurite orientation (anterograde to right) in motor axons, neuromuscular synapse terminals and Purkinje cell dendrites (n≥9 neurites from ≥3 mice for each group). (e) Mean frequency of comet orientations colour-binned for anterograde and retrograde orientations (n≥10 neurites from ≥3 mice for each group). Scale bar ina,b, 5 μm. 1 and Supplementary Table 1 ). For all experiments, the mouse line with the lowest expression level and a punctate pattern of fluorescence was used (line J045 for most experiments; J023 for cortical imaging), as strong overexpression of EB3 leads to binding to the entire microtubule lattice [18] and pathological swellings in some axons (for example, line J030, which we did not use in our experiments). To further estimate the level of overexpression of EB3-YFP compared with endogenous EB3, we performed single-cell PCR on EB3-YFP-positive and -negative Purkinje cells, of which only a subset is labelled in line J045. In heterozygous animals of this low-expressing line, YFP-positive cells show a threefold increase in messenger RNA compared with YFP-negative Purkinje cells (ΔCp=1.57, n =26 versus 11 cells per 3 animals). In line with these results, the transgene did not cause any obvious changes of the behaviour, lifespan or fertility of the mice and did not affect neuromuscular morphology, posttranslational tubulin modifications, axonal transport or ultrastructure ( Supplementary Figs 2 and 3 ). Moreover, when we isolated adult dorsal root ganglionic (DRG) and embryonic hippocampal neurons from Thy1 :EB3-YFP mice (J045 line), we found that the characteristics of transgene-based labelling matched those seen in classical transfection-based assays [10] , that transgene-based labelling co-localized with labelling derived from a spectrally distinct transfected construct, and densities of endogenous accumulations of another EB (EB1) were not affected by the presence of the EB3-YFP transgene ( Supplementary Fig. 4 ). Together, these controls show that in Thy1 :EB3-YFP mice expression of the transgene is largely non-toxic and inert as previous established in vitro [10] , [18] . Microtubule dynamics in different neuronal compartments To explore whether Thy1 :EB3-YFP mice allowed visualizing dynamic microtubules in intact, mature neurites, we used high-resolution time-lapse microscopy of peripheral axons in intercostal nerves of triangularis sterni explants [19] . We found that the transgenic fusion protein revealed the tips of microtubules as a dynamic pattern of ‘comet-like’ structures against a faint background of cytoplasmic labelling ( Fig. 1 and Supplementary Movie 1 ). Recordings in the sciatic nerves of anesthetized mice in vivo [15] showed a similar pattern ( Fig. 2a,b and Supplementary Movie 2 ). Determining the density of these comets ex vivo and in vivo thus provided a direct measure of the local dynamics of the microtubule cytoskeleton in myelinated axons ex vivo (0.065±0.002 comets μm −2 axonal area in distal motor axons, n =32 axons per 8 animals; 0.025±0.001 μm −2 in proximal intercostal axons, n =27/6; mean±s.e.m. ; for reasoning behind two-dimensional analysis, see Methods) and in vivo in the sciatic nerve (0.042±0.005 μm −2 , measured at mid-thigh level, an intermediate proximal–distal position, n =15/3; mean±s.e.m.). EB3-YFP comets appeared suddenly, propagated for a distance of a few microns and disappeared (speed: 0.112±0.003 μm s −1 in distal axons ex vivo ; n =32/8; mean±s.e.m.). While the speed in mature axons was found to be lower than reported in vitro and in invertebrates (for example, 0.22 μm s −1 in hippocampal cultures [10] ), other comet characteristics, such as orientation and length, are conserved across models. A more detailed analysis of different phases of microtubule growth requires increased imaging frequency [20] , [21] , for example, 2 Hz instead of our routine acquisition rate of 0.5 Hz. As shown previously in vitro [20] , such an imaging regime allows distinguishing growth, pause and reset (likely depolymerization) phases along individual microtubule tracks ( Supplementary Fig. 5 ). However, because high-frequency imaging leads to faster photo-bleaching, we performed the subsequent experiments at 0.5 Hz, which is sufficient to analyse changes in microtubule orientation and density. Figure 1: Imaging microtubule dynamics in Thy1 :EB3-YFP mice. ( a ) A neuromuscular junction (postsynaptic receptors labelled with fluorescently tagged Bungarotoxin, red) and terminal motor axons in an acute Thy1 :EB3-YFP triangularis sterni explant. Inset shows eight frames cropped (dashed box in main panel) from a time-lapse sequence of this area highlighting an anterogradely directed EB3 comet (pseudocolored in green). The main panel shows a maximum intensity projection of 20 s within the time lapse (for full movie, see Supplementary Movie 1 online), where each comet is represented by a colour-coded arrow (anterograde, green; retrograde, blue). ( b ) Dendrite of a Purkinje cell in an acute cerebellar slice represented in the same way as in ( a ) (see Supplementary Movie 3 ). Note the more frequent occurrence of retrogradely directed comets. ( c ) Comet density in different neuronal compartments ( n ≥10 neurites from ≥3 mice for each group; horizontal line shows mean±s.e.m.). ( d ) Polar plots (that is frequency histograms with angular orientation shown in a circle) of comet directionality in relation to neurite orientation (anterograde to right) in motor axons, neuromuscular synapse terminals and Purkinje cell dendrites ( n ≥9 neurites from ≥3 mice for each group). ( e ) Mean frequency of comet orientations colour-binned for anterograde and retrograde orientations ( n ≥10 neurites from ≥3 mice for each group). Scale bar in a , b , 5 μm. 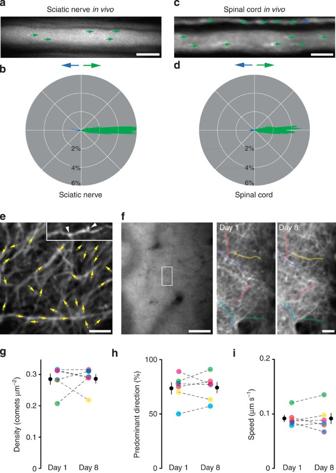Figure 2:In vivoimaging of microtubule dynamics in the PNS and CNS. (a) Microtubule dynamics in a sciatic nerve axon of an anesthetizedThy1:EB3-YFP mouse (image represented as inFig. 1; seeSupplementary Movie 2). (b) Polar plot shows comet directionality of axons in the sciatic nerve. (c) Microtubule dynamics in an axon in the lumbar spinal cordin vivo(seeSupplementary Movie 4). (d) Polar plot of axons in lumbar spinal cord. (e) Neurites of the somatosensory cortex imaged through a cranial windowin vivo(seeSupplementary Movie 5). Comets are colour coded in yellow, as anterograde and retrograde cannot always be defined in this preparation. Inset shows CFP channel of another mouse that was injected with a CFP-expressing adeno-associated virus to illustrate spine-like protrusions (arrowheads) on EB3-measured neurites. (f) Chronic imaging of the same neurites in the somatosensory cortexin vivoover 1 week. A larger overview of the cranial window (left) allows the same six neurites to be identified on day 1 and 8 (boxed on the left; neurites pseudocolored on the right). (g,h,i) Density, predominant direction and speed were measured in the same six neurites (identified by colour and linked by dashed line; black data symbol shows mean±s.e.m.) as shown in (f) on day 1 and day 8. Scale bar ina,b,e,f(higher magnification panels and inset) 5 μm and inf(overview) 50 μm. Full size image Figure 2: In vivo imaging of microtubule dynamics in the PNS and CNS. ( a ) Microtubule dynamics in a sciatic nerve axon of an anesthetized Thy1 :EB3-YFP mouse (image represented as in Fig. 1 ; see Supplementary Movie 2 ). ( b ) Polar plot shows comet directionality of axons in the sciatic nerve. ( c ) Microtubule dynamics in an axon in the lumbar spinal cord in vivo (see Supplementary Movie 4 ). ( d ) Polar plot of axons in lumbar spinal cord. ( e ) Neurites of the somatosensory cortex imaged through a cranial window in vivo (see Supplementary Movie 5 ). Comets are colour coded in yellow, as anterograde and retrograde cannot always be defined in this preparation. Inset shows CFP channel of another mouse that was injected with a CFP-expressing adeno-associated virus to illustrate spine-like protrusions (arrowheads) on EB3-measured neurites. ( f ) Chronic imaging of the same neurites in the somatosensory cortex in vivo over 1 week. A larger overview of the cranial window (left) allows the same six neurites to be identified on day 1 and 8 (boxed on the left; neurites pseudocolored on the right). ( g , h , i ) Density, predominant direction and speed were measured in the same six neurites (identified by colour and linked by dashed line; black data symbol shows mean±s.e.m.) as shown in ( f ) on day 1 and day 8. Scale bar in a , b , e , f (higher magnification panels and inset) 5 μm and in f (overview) 50 μm. Full size image To gain further insight into local cytoskeletal properties, we investigated the orientation of dynamic microtubules in different neuronal compartments. In distal intercostal axons, the vast majority (95±1%, n =32/8; mean±s.e.m.) of dynamic microtubules have a ‘plus-end out’ polarity ( Fig. 1 ); the properties of dynamic microtubules in neuromuscular presynaptic terminals appeared similar, albeit comet density was higher and orientation less stringent (density: 0.118±0.007 μm −2 ; ‘plus-end out’ orientation: 83±3%; n =13/4; mean±s.e.m.). In contrast, when we imaged microtubule dynamics in proximal Purkinje cell dendrites in acute cerebellar slices, we found a very dense (0.141±0.011 μm −2 ; n =10/3; mean±s.e.m.) pattern of comets of mixed orientation (‘plus-end out’ orientation: 65±4%; mean±s.e.m. ; in line with previous reports in cell culture [10] , [22] ; Figure 1b–e and Supplementary Movie 3 ). To confirm that the reported differences were indeed related to the imaged compartment, rather than a spurious effect of explanting CNS tissue, we devised two-photon imaging assays to measure microtubule dynamics in individual spinal axons and in cortical neurites of live anesthetized mice ( Fig. 2a–d , Supplementary Movies 4 and 5 ). The in vivo density of dynamic microtubules in the spinal cord (0.033±0.002 μm −2 ; n =15/3; mean±s.e.m.) was in a similar range to what we measured in the explanted intercostal nerves and in the sciatic nerve in vivo . Also microtubule orientation (‘plus-end out’: 93±1; n =15/3; mean±s.e.m.) and comet speed (0.147±0.004 μm s −1 ; n =15/3; mean±s.e.m.) were comparable to previous measurements. To image microtubule dynamics in vivo in the brain, we implanted chronic cranial windows [23] , [24] , which allowed acquiring time-lapse movies of neurons from the somatosensory cortex in adult Thy1 :EB3-YFP transgenic mice (Line J023). Despite movement artifacts and reduced signal-to-noise levels in these recordings, we were able to measure density (0.222±0.017 μm −2 ; n =18/5), speed (0.101±0.004 μm s −1 ; n =18/5) and predominant orientation (73±4; n =18/5; all mean±s.e.m.) of dynamic microtubules in individual cortical neurites ( Fig. 2e and Supplementary Movie 5 ). Most of the imaged neurites are likely dendritic processes, as confirmed by injection of an adeno-associated virus expressing cytoplasmic CFP, which reveals the presence of spine-like protrusions ( Fig. 2e ). This in vivo imaging paradigm also allowed longitudinal assessment of microtubule behaviour over periods of 7 days ( Fig. 2f ). Under physiological conditions, the parameters of dynamic microtubules did not change over time ( n =8/2; Fig. 2g–i ), confirming that our assay provides a robust baseline for future in vivo assessment of microtubule changes in plasticity paradigms. In summary of these in vivo experiments, we can conclude that axons show a lower density of stringently oriented dynamic microtubules compared with dendrites, where densities are higher, but orientation more variable. Moreover, along axons there appears to be a proximal-to-distal gradient of increasing density but lower orientation stringency of comets. Finally, most parameters of microtubule dynamics appear insensitive to acute isolation (provided the imaging site stays clear of any axon transection site, see below), stable over time and comparable between PNS and CNS. As the ease of recording, and the stability and quality of measurements are superior in ex vivo nerve–muscle explants compared with the in vivo setting, we used the explant for subsequent experiments. Microtubule dynamics under pathological conditions Next, we asked whether our assay could provide useful information in the context of disease-related alterations of the microtubule cytoskeleton. Microtubules play central roles in dynamic cellular processes, such as mitosis, but also under homeostatic conditions, for example by providing stability and support. Both functions of microtubules have been targeted pharmacologically, which comes at risk of substantial side effects. For example, high doses of microtubule-stabilizing drugs, such as paclitaxel [25] , are used as cytostatic agents in oncology, but their application is limited by the risk of inducing toxic neuropathies [26] . Paradoxically, at low doses, paclitaxel and related drugs are also considered as potential therapeutic agents to promote axon survival, as microtubule stabilization might protect axons after trauma [27] , [28] and against degeneration [6] , [7] , [29] . Obviously, the double-edged effect of microtubule-stabilizing drugs on axons means that it is paramount to devise precise dosing schemes and understand their cell biological consequences. Hence, an assay that allows direct monitoring of the effects of microtubule-stabilizing drugs would be of considerable use. To explore this, we performed dose–response studies to see at which concentration paclitaxel affects dynamic microtubules in intact myelinated axons. Time-lapse recordings of Thy1 :EB3-YFP intercostal axons revealed loss of EB3 comets after high paclitaxel doses (EC 50 at 60 min≈2 μM; Fig. 3a,b ), suggesting ‘freezing’ of microtubule dynamics. In contrast, at low paclitaxel doses (≤1.5 μM) EB3 comets were partially preserved for at least 3 h. To probe whether such in situ dosing would allow predictions about outcomes that favoured axon preservation or loss, we explored the effects of different paclitaxel doses on acute axonal degeneration (AAD [30] ). AAD removes parts of severed axons within an hour of axotomy and has been previously identified as a possible target for low-dose paclitaxel therapy [27] . Indeed, when we measured the extent of AAD-mediated axonal dieback after two-photon laser cuts of motor axons, we found a significant protection of the axons at low doses (1.5 μM) of paclitaxel ( Fig. 3c,d ), while high paclitaxel doses (10 μM) exacerbated axonal dieback. 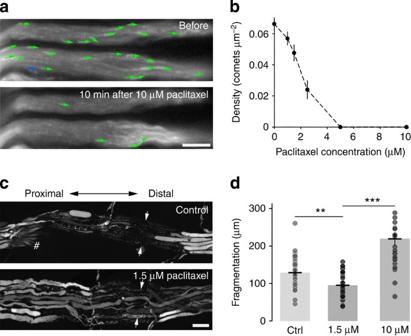Figure 3: Microtubule dynamics after exposure to paclitaxel. (a,b) The microtubule-stabilizing drug paclitaxel leads to a dose-dependent loss of comets in motor axonsex vivo. (a) shows time-lapse analysis represented as inFig. 1; in (b), the corresponding dose–response curve measured 60 min after paclitaxel application (n≥11 axons from 3 mice for each group; mean±s.e.m.). (c,d) Low-dose paclitaxel protects against acute axonal degeneration (AAD). (c) Shows confocal micrographs of axon fascicles in explants fromThy1:YFP-16 mice (all motor axons are labelled), 1 h after several axons were severed by two-photon microsurgery (arrows) in untreated (top) and paclitaxel-pretreated (1.5 μM for 1.5 h before and for 1 h after axotomy; bottom) explants. Note dieback marked by trails of axon fragments. Some axons could not be severed as they lay too deep (asterisk); other axons leave the nerve in a fascicle (pound symbol); both were not included in the analysis. (d) Shows a quantification of the AAD-mediated dieback distance in untreated control, 1.5 and 10 μM paclitaxel-treated axons (n≥25 axons from 3 mice per group horizontal line shows mean±s.e.m.). Scale bar ina5 μm and inc20 μm. ***P<0.001; **P<0.01,t-test. Figure 3: Microtubule dynamics after exposure to paclitaxel. ( a , b ) The microtubule-stabilizing drug paclitaxel leads to a dose-dependent loss of comets in motor axons ex vivo . ( a ) shows time-lapse analysis represented as in Fig. 1 ; in ( b ), the corresponding dose–response curve measured 60 min after paclitaxel application ( n ≥11 axons from 3 mice for each group; mean±s.e.m.). ( c , d ) Low-dose paclitaxel protects against acute axonal degeneration (AAD). ( c ) Shows confocal micrographs of axon fascicles in explants from Thy1: YFP-16 mice (all motor axons are labelled), 1 h after several axons were severed by two-photon microsurgery (arrows) in untreated (top) and paclitaxel-pretreated (1.5 μM for 1.5 h before and for 1 h after axotomy; bottom) explants. Note dieback marked by trails of axon fragments. Some axons could not be severed as they lay too deep (asterisk); other axons leave the nerve in a fascicle (pound symbol); both were not included in the analysis. ( d ) Shows a quantification of the AAD-mediated dieback distance in untreated control, 1.5 and 10 μM paclitaxel-treated axons ( n ≥25 axons from 3 mice per group horizontal line shows mean±s.e.m.). Scale bar in a 5 μm and in c 20 μm. *** P <0.001; ** P <0.01, t -test. Full size image Previous studies in invertebrate neurons have suggested that axotomy has drastic acute and chronic effects on microtubule dynamics [11] , [31] . To what degree such findings also hold true in mature mammalian axons remains unclear, as non-mammalian axons differ substantially from mammalian ones in their behaviour after injury [32] , [33] . Our assay revealed that immediately (<5 min) after laser transection of motor axons [34] , a greater than fourfold increase in dynamic microtubule density was observed compared with non-severed axons (at 0–10 μm from the axon-end: 0.283±0.032 μm −2 axonal area; n =9/7; mean±s.e.m. ; Fig. 4a,b , Supplementary Movie 6 ). This increase was a local phenomenon, as comet density remained normal 60–70 μm proximal to the injury site. The polarity of comets in the area proximal to the cut was largely unaltered, with the majority of the excess comets propagating anterogradely, although the orientation of individual comets paralleled the axonal axis less strictly near the severed end than further away. While our results confirm acute injury-induced changes in microtubule dynamics, we did not observe ‘traps’ of microtubules that are directed in opposing directions as described in transected axons of isolated Aplysia neurons [11] . 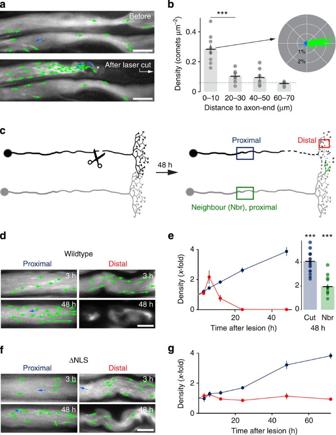Figure 4: Microtubule dynamics after acute and chronic injury. (a,b) Acute axotomy by two-photon laser (axotomy site outside of the frame; arrow ina) induces a rapid increase in comet density at the proximal axon-end (asterisk;Supplementary Movie 6). Comet density in the lower axon is unchanged, because the cut is>60 μm outside of the frame. Quantification (b) shows that this effect is confined to within less than 60 μm from the axon-end and comet orientation is largely unaltered (horizontal line shows mean±s.e.m.; polar plot of the 0–10 μm segment shown as insert; the dashed green line indicates control values;n≥7 neurites from ≥5 mice for each group; polar plot from four axons from four mice). (c–e) In contrast to the local increase in microtubule dynamics seen acutely after axotomy, global changes in comet density are found within 12 h after nerve cut (schematic of experiment and measurement sites inc). The ‘neighbour’ is an uncut adjacent nerve that can sprout into the denervated territory (green sprout symbol on the right inc). Proximal of the cut (~1 mm away) comet density steadily increases, while distally an initial spike in dynamics is followed by a decline before fragmentation (d,e, left). (e) Right shows that axons in the neighbouring nerve that are not cut, but receive a growth stimulus (‘Nbr’), also show increased microtubule dynamics after 48 h (n≥10 neurites from ≥3 mice for each condition; bar showing ‘cut, 48 h’ is a re-plot from time course on left; horizontal line and data symbols show mean±s.e.m., respectively). (f,g) Changes in microtubule dynamics in the distal axotomized stump are abolished by overexpressing a fusion protein that blocks Wallerian degeneration (‘ΔNLS’), while the proximal changes are delayed but still present (n≥11 neurites from ≥2 mice for each group; data symbols indicate mean±s.e.m.). In panelse,gsome error bars are hidden by the data symbol. Scale bar in all panels 5 μm. ***P<0.001, analysis of variance. Figure 4: Microtubule dynamics after acute and chronic injury. ( a , b ) Acute axotomy by two-photon laser (axotomy site outside of the frame; arrow in a ) induces a rapid increase in comet density at the proximal axon-end (asterisk; Supplementary Movie 6 ). Comet density in the lower axon is unchanged, because the cut is>60 μm outside of the frame. Quantification ( b ) shows that this effect is confined to within less than 60 μm from the axon-end and comet orientation is largely unaltered (horizontal line shows mean±s.e.m. ; polar plot of the 0–10 μm segment shown as insert; the dashed green line indicates control values; n ≥7 neurites from ≥5 mice for each group; polar plot from four axons from four mice). ( c – e ) In contrast to the local increase in microtubule dynamics seen acutely after axotomy, global changes in comet density are found within 12 h after nerve cut (schematic of experiment and measurement sites in c ). The ‘neighbour’ is an uncut adjacent nerve that can sprout into the denervated territory (green sprout symbol on the right in c ). Proximal of the cut (~1 mm away) comet density steadily increases, while distally an initial spike in dynamics is followed by a decline before fragmentation ( d , e , left). ( e ) Right shows that axons in the neighbouring nerve that are not cut, but receive a growth stimulus (‘Nbr’), also show increased microtubule dynamics after 48 h ( n ≥10 neurites from ≥3 mice for each condition; bar showing ‘cut, 48 h’ is a re-plot from time course on left; horizontal line and data symbols show mean±s.e.m., respectively). ( f , g ) Changes in microtubule dynamics in the distal axotomized stump are abolished by overexpressing a fusion protein that blocks Wallerian degeneration (‘ΔNLS’), while the proximal changes are delayed but still present ( n ≥11 neurites from ≥2 mice for each group; data symbols indicate mean±s.e.m.). In panels e , g some error bars are hidden by the data symbol. Scale bar in all panels 5 μm. *** P <0.001, analysis of variance. Full size image To examine whether more global changes of microtubule dynamics occur at a later stage of the injury response as shown in flies [35] , we mechanically transected intercostal nerves in vivo [15] and then imaged EB3-YFP dynamics distal and proximal to the lesion between 3 h and 2 days after injury ( Fig. 4c–e ). A global proximal increase in comet density started 6 h after cut and reached a greater than threefold increase within 2 days (at ~1 mm from the lesion, 6 h after cut: 0.033±0.003 versus 0.023±0.002 μm −2 in uncut contralateral control nerves; 2 days after cut: 0.087±0.006 versus 0.022±0.001 μm −2 ; n ≥9/2 for both time points; all mean±s.e.m.). After transection, motor axons start to form growing tips to reinnervate their target muscle [36] . When we measured microtubule dynamics in axon tips during regeneration, we detected a significant sustained increase in dynamic microtubule densities (9 days after cut: 0.195±0.020; n =15/3; mean±s.e.m. ; Supplementary Movie 7 ). Surprisingly, comet density also increased transiently in the distal nerve stump 6 h after injury, but decreased before Wallerian fragmentation set in ( Fig. 4d,e ). To ascertain whether this distal increase was part of the Wallerian degeneration programme [37] , even though it preceded overt fragmentation by several hours, we crossed Thy1 :EB3-YFP transgenic animals with Δ NLS-Wld S mice that express a predominantly axonal and therefore particularly potent version (deleted nuclear localization signal; ΔNLS) of the slow Wallerian degeneration (Wld S ) protein [38] . In such mice, the distal stump of cut axons remains intact for up to 2 weeks. While the proximal response to axotomy was similar to the wild-type situation, although the increase in comet density was somewhat delayed, the distal stump showed largely unaltered comet densities at all time points examined after injury (up to 3 days; Fig. 4f,g ). This suggests that the proximal and the distal increase in comet densities are mechanistically distinct and that changes in microtubule dynamics are immediately linked to the Wallerian degeneration programme in disconnected axon segments. So, on the one hand, increased microtubule dynamics could serve as a tag of destabilized axons that are destined to degenerate. On the other hand, the delayed and sustained increase in microtubule dynamics in the proximal stump correlates with regenerative growth, rather than with degeneration. We therefore wondered, whether microtubule remodelling could also be found in axons that receive growth-promoting stimuli, but were never injured. As the triangularis muscle is intersegmental and receives input from several intercostal nerves [19] , axotomy of one intercostal nerve can induce expansion of motor units in neighbouring nerves, as their axons strive to reinnervate vacated neuromuscular junction sites ( Fig. 4c ). Indeed, when we assayed microtubule dynamics in neighbouring, non-transected intercostal axons, we found that comet density doubled (2 days after cut: 0.042±0.004; n =15/3 versus contralateral side: 0.020±0.001; n =10/3; all mean±s.e.m. ; Fig. 4e , right). These results suggest that EB3-comet density could serve as a general marker of ongoing or imminent remodelling of axonal arbours. The drastic changes in microtubule dynamics that we found in traumatic forms of axon degeneration in Thy1 :EB3-YFP mice raised the question of whether similar changes can be found in chronic neurodegenerative diseases [6] . To investigate this, we crossed Thy1 :EB3-YFP mice to mice that overexpress mutant forms of human superoxide dismutase 1 (SOD mice), a widely used model of familial amyotrophic lateral sclerosis. Indeed, in two different strains of SOD mice (for description of mutants, see ref. 39 ), showing either a very rapid (SOD1 G93A ) or a more protracted (SOD1 G85R ) disease course, we found an increase in comet density in otherwise intact looking intercostal axons. In contrast, 4-month-old control mice that overexpressed a non-mutated form of human SOD1 showed normal microtubule dynamics ( Fig. 5 ). 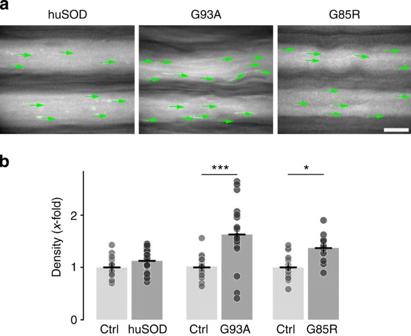Figure 5: Microtubule dynamics in neurodegenerative disease. (a,b) Microtubule dynamics are altered with increased comet densities in two models of familial ALS, but not in control mice that overexpress a non-mutated form of human SOD1 (Ctrl: respective wild-type litter mates as controls; ‘huSOD’, non-mutated form of SOD1, P120; ‘G93A’: SOD1G93Amutation, P120; ‘G85R’, SOD1G85Rmutation, preterminal;n≥10 neurites from ≥2 mice for each group; data symbols indicate mean±s.e.m.). Scale bar in (a) 5 μm. ***P<0.001; *P<0.05, analysis of variance. Figure 5: Microtubule dynamics in neurodegenerative disease. ( a , b ) Microtubule dynamics are altered with increased comet densities in two models of familial ALS, but not in control mice that overexpress a non-mutated form of human SOD1 (Ctrl: respective wild-type litter mates as controls; ‘huSOD’, non-mutated form of SOD1, P120; ‘G93A’: SOD1 G93A mutation, P120; ‘G85R’, SOD1 G85R mutation, preterminal; n ≥10 neurites from ≥2 mice for each group; data symbols indicate mean±s.e.m.). Scale bar in ( a ) 5 μm. *** P <0.001; * P <0.05, analysis of variance. Full size image Taken together, our study demonstrates that in vivo imaging of Thy1 :EB3-YFP mice allows assaying microtubule dynamics and polarization in different compartments of fully mature mammalian neurons in the PNS and CNS. Thus, the status of the microtubule cytoskeleton can be determined in acute and chronic models of axonal injury, as well as under the influence of microtubule-modifying drugs, which are in wide use in oncology as cytostatic agents where neurotoxicity limits their use [26] . Moreover, modulating microtubule stability has been suggested as a therapeutic approach to prevent secondary axon loss after trauma, promote regrowth or even halt neurodegeneration [7] , [28] . Importantly, it is not always clear to what extent such beneficial effects result from direct action on neurons or rather on other cells, such as glia or fibroblasts. As dosing and cell specificity are clearly critical in clinical translation, our neuron-specific in vivo assay will be useful in further developing such approaches in mammals. Finally, increased microtubule dynamics might serve as an early indicator of axon destabilization and plasticity, as it equally precedes degenerative destruction (in Wallerian degeneration or in amyotrophic lateral sclerosis models), as well as denervation-induced outgrowth. Given that microtubule dynamics also marks a subset of dendritic spines and regulates spine shape in vitro [40] , increased EB3-comet activity could serve as a tag of remodelling neurite segments. Clearly, final proof of this notion will require careful in vivo experiments, for example, using induced remodelling paradigms in the somatosensory cortex [41] or spontaneous remodelling processes, such as those found in developing motor axons [42] . Importantly, with the new in vivo tools presented here, testing this hypothesis, as well as exploring the role of microtubule remodelling in a broad range of mouse models of neurological diseases is now possible. Still, before our approach is transferred to new applications, some considerations need to be kept in mind: First, in Thy1 :EB3-YFP mice, a biologically active fusion protein is overexpressed. As even YFP overexpression alone can have toxic effects in axons [43] , it is important to include appropriate controls in any new setting in which the assay is used. Importantly, in our low-expressing mouse lines overexpression seems moderate, and so far, we did not detect any signs of pathology. Furthermore, for those parameters that can be compared, our assay is in accordance with previous approaches (for example, comet-like versus filamentous distribution; coincidence of transgene- and transfection-based labelling in vitro ; microtubule orientation [8] , [10] , [44] ). In addition to general toxicity, specific effects of EB3 overexpression should be considered. For example, EB3 interacts with other plus-end-binding proteins, such as CLIPs [18] . Our construct lacks this interaction domain [10] ; however, as the endogenous EB3 locus is intact, only a partial loss of function would be expected—and indeed, in vitro this interference becomes relevant only at high levels of overexpression that coincide with loss of a comet-like staining pattern [18] . Second, CNS in vivo imaging of microtubule dynamics requires careful design of excitation and emission optics of the two-photon system—which is not surprising given that the structure imaged here has a size roughly an order of magnitude below the diffraction limit in width (a microtubule’s diameter is ~25 nm) and which has an intrinsic limitation in ‘signal-over-background’ if high levels of overexpression are avoided. Therefore, for automated analysis as previously established for EB comets in vitro [20] , even optimally acquired in vivo data sets can prove challenging. Third, while EB3-YFP marks a well-defined structure in cell biological terms, an increase in comet density alone does not directly predict whether the microtubule cytoskeleton undergoes net expansion or contraction, as dynamic microtubules would be expected to be more abundant in both settings. However, microtubular breakdown and expansion are linked to early steps of neurite loss and outgrowth, respectively, so that our assay provides a means to identify sites of imminent neuronal remodelling. Hence, while above-mentioned considerations are important to keep in mind for future applications, the assay described here adds microtubule remodelling to the growing list of cell biological properties of neurons that can be measured in vivo in the mammalian nervous system during development, homeostasis and disease. Animals For specific labelling of dynamic microtubule tips in neurons, we used regulatory elements of the Thy1 -promoter [14] to express YFP-tagged end-binding protein 3 (EB3) in neurons [45] . For this, an amino-terminal in-frame fusion was generated between the coding sequence of YFP and EB3 (derived from an EB3-GFP vector provided by B. Link, Medical College of Wisconsin, USA). This EB3-YFP fusion gene was cloned into an expression vector downstream of neuron-specific elements of the Thy1 -promoter [14] , [46] . Thy1: EB3-YFP transgenic mice were generated using standard pronuclear injection procedures, and 10 founder lines were screened to establish the three transgenic mouse strains (J045, J023 and J030) described in this study—these are now past the F7 generation and appear to be stable in their expression pattern. J045, the lowest expressing line, was used for most experiments. Parameters of neuromuscular health were determined in J045, as well as J023, to ensure that also higher levels of EB3 expression had no detrimental effects. J030 showed overexpression effects and was not further used. MitoMice [15] (transgenic mice with CFP-labelled neuronal mitochondria to measure mitochondrial transport), Thy1 :YFP-16 mice [14] (which express cytoplasmic YFP in all motor axons) and ΔNLS-Wld S mice [38] (transgenic mice expressing the ‘Wallerian degeneration slow’ fusion protein carrying two-point mutations in a nuclear localization signal that redistribute the gene product to the cytoplasm; provided by M. Coleman, Babraham Institute, Cambridge, UK) were previously published. Mice overexpressing human superoxide dismutase 1 (wild type, G93A [47] and G85R [48] mutations) were obtained from The Jackson Laboratory, Bar Harbor, USA. ‘Preterminal’ G85R animals had lost 10% of their peak body weight and were unable to sustain their body weight hanging from a grid for >30 s [39] . Male and female animals were used, ranging in age from 6 to 18 weeks. All animal work conformed to institutional and national guidelines. Single-cell reverse transciptase PCR For collection of Purkinje cell cytoplasm we slightly modified a previously described protocol [49] . In brief, slices were placed in a recording chamber and perfused with artificial cerebrospinal fluid at room temperature. Purkinje cells were identified visually using an upright microscope (Eclipse E600FN; Nikon). Patch clamp pipettes were made from borosilicate glass (2.0/0.3 mm) using a Narishige PC-10 pipette puller. Tip diameters of about one-third of the cell soma diameter (8 μm for Purkinje cells) were produced by modifying the heat of the second pulling step. The pipette solution consisted of 4 μl H 2 O and 1 μl M-MLV reverse transcriptase 5 × reaction buffer (‘First Strand Buffer’, FSB; Promega). Under visual control, the tip of the pipette was gently attached to the selected cell and the soma sucked in. Under a dissecting microscope, the content of the pipette was pressure-ejected into a 0.5 ml reaction tube and frozen at −80 °C. Reverse transcription was performed as follows: The collected material was complemented with ‘Master Mix 1’ (1 μl 1% Nonidet P-40 and 1 μl 5 mM random primers p(dN)6, Roche; 1 μl 10 mM of each dNTPs, 1 μl FSB and 1 μl RNasin plus; Promega), incubated at 70 °C and then at 0 °C, 5 min each. Ten microlitres of ‘Master Mix 2′ (2 μl FSB, 6.5 μl H2O and 1.5 μl M-MLV reverse transcriptase; Promega) were added, followed by incubation for 1–2 h at 37 °C. The resulting cDNA was purified using silica matrix and stored at −80 °C. For the comparison of expression levels in individual cells, 80% of cDNA material of a single cell was used. Rapid cycle PCR reactions performed in 20 μl reactions in glass capillaries according to the manufacturer’s instructions using the LightCycler FastStart DNA Master SYBR Green I kit (Roche). The amount of primer used per reaction was 10 pmol, the concentration of MgCl2 was 3 mM. Rapid cycle reverse transciptase PCR was performed on the LightCycler (Roche) and analysed with the LightCycler analysis software (version 3.5.3) in the log-linear phase using the so called ‘fit point’ method [49] . Cell culture Dorsal root ganglia were cultured following a published protocol [50] . Briefly, the ganglia from L4, L5 and L6 spinal levels of adult (>2 month old) Thy1 :EB3-YFP transgenic mice were dissected and incubated at 37 °C in 3% collagenase type I (3,000 U ml −1 , Worthington Biochemical) for 45 min. The ganglia were then digested at 37 °C with 0.25% trypsin (Roche) for 15 min. By adding DMEM/10% horse serum, the reaction was stopped, and cells collected by centrifugation at 700 r.p.m. for 5 min. Cells were resuspended in NeuroBasal media complemented with B-27 supplement, L -glutamine and penicillin–streptomycin (all Invitrogen) and plated on poly- L -lysine- (PLL; 1 mg ml −1 , Sigma) and laminin (5 μg ml −1 , Roche)-coated glass coverslips or glass-bottom dishes (MatTek). Cells were kept at 37 °C in a humidified atmosphere containing 5% CO2. Primary hippocampal neurons derived from embryonic (E17) C57BL/6JCrl wild type (Charles River) or Thy1 :EB3-YFP transgenic mice were cultured as established in previous studies [51] . In brief, hippocampi were dissected, digested with 0.05% trypsin-EDTA (Invitrogen) and washed with Hank’s balanced salt solution. Afterwards cells were triturated using Pasteur pipettes and plated on PLL (Sigma)-coated coverslips or glass-bottom dishes in MEM/10% horse serum. After 4 h, media was changed to MEM containing N2 supplements. Neurons were transfected using the Nucleofector system (Amaxa). The EB3-mCherry and EB3-GFP plasmids were purified using the EndoFree Maxiprep Kit, (Qiagen) and used at a concentration of 3 μg. Microtubule dynamics of either Thy1 :EB3-YFP transgenic or EB3-mCherry/-GFP-transfected wild-type cells were analysed 8 h or 24 h after plating. To this end, fluorescent images with a pixel size of 0.106 μm were acquired in 3-s intervals for 3 min using a DeltaVision RT setup. Videos with 7 frames per second were processed using the open-source software, ImageJ/Fiji. Tissue preparation, immunohistochemistry and microscopy For tissue analysis, mice were transcardially perfused with 4% paraformaldehyde (PFA) diluted in 0.01 M phosphate-buffered saline (1 × PBS) and post fixed for 24 h in 4% PFA in 1 × PBS. Following dissection, the tissue of interest (brain, spinal cord and eye) was either prepared for cryo-sectioning by incubation in 30% w/v sucrose (Sigma) in 1 × PBS or vibratome sectioned. Sections (thickness: 30 μm for cryostat, 100 μm for vibratome) were stained with Neurotrace 594 (Molecular Probes, diluted 1:500 in 1 × PBS) to label cell bodies and nuclei. Sections were mounted in Vectashield (Vector Laboratories) and image stacks were recorded using an FV1000 confocal microscope (Olympus) equipped with × 20/0.8 N.A. and × 60/1.42 N.A. oil-immersion objectives. Images were processed using ImageJ/Fiji and Adobe Photoshop. Triangularis sterni muscles were fixed in methanol (−20 °C) for 10 min, and then for 1 h in 4% PFA, stained with Alexa594-conjugated α-Bungarotoxin (Invitrogen, 50 mg μl −1 diluted 1:50 in 1 × PBS) and Alexa647-conjugated phalloidin (Invitrogen, 200 units ml −1 methanol, diluted 1:50 in 1 × PBS) to visualize acetylcholine receptors at the neuromuscular junction or muscle fibres, respectively, and analysed by confocal microscopy for parameters of neuromuscular health. Some muscles were stained with tubulin antibodies (Alexa555-conjugated mouse anti-β-tubulin, BD Pharmingen; anti-glu-α-tubulin mouse monoclonal, Synaptic Systems) using standard protocols. Electron microscopy Animals were perfused transcardially with 2.5% glutaraldehyde and 2% PFA in 0.1 M PBS. After post fixation for 24 h, nerves were isolated and stained with 1% osmium tetroxide reduced in 1.5% potassium ferrocyanide. Tissues were washed in four changes of 0.1 M sodium cacodylate buffer, dehydrated in an ascending ethanol series and two changes of 100% propylene oxide, infiltrated with Araldite 502/EMbed812 resin (Electron Microscopy Sciences), and finally polymerized at 60 °C for 48 h. Tissue blocks were oriented to cut either cross or lateral ultrathin sections (~60 nm). Sections were collected on pioloform-coated slot grids and stained with 2% uranyl acetate and Reynold’s lead citrate. Electron micrographs were obtained with a JEM-1400 transmission electron microscope (JEOL) operating at 120 kV. Micrographs were collected with an Ultrascan 1000 camera (Gatan) at a resolution of 1.6 nm per pixel. Imaging microtubule dynamics ex vivo and in vivo For the triangularis sterni explant, mice were lethally anesthetized with isoflurane and the anterior thoracic wall (with the attached triangularis sterni muscle and its innervating intercostal nerves) was isolated by cutting the ribs close to the vertebral column. The explant was pinned down on a Sylgard-coated 3.5 cm plastic Petri dish using minutien pins (Fine Science Tools). After excision, explants were kept in 95% O 2 / 5% CO 2 -bubbled Ringer's solution (125 mM NaCl, 2.5 mM KCl, 1.25 mM NaH 2 PO 4 , 26 mM NaHCO 3 , 2 mM CaCl 2 , 1 mM MgCl 2 , 20 mM glucose). During imaging, explants were kept on a heated stage (33–36 °C; in this range, comet density varied by less than 20%; data not shown) with a slow and steady flow of warmed and oxygenated Ringer’s solution [19] . ‘Proximal’ are recording sites in the intercostal nerve proper; ‘distal’ are sites beyond the entry point of axons into the muscle. For in vivo imaging, the sciatic nerve was exposed in anesthetized mice (1.5% ketamine, 0.1% vol/vol xylazine intraperitoneally) as described previously [15] , and imaged as described below. Animals were euthanized at the end of the experiment by cervical dislocation in deep anaesthesia. Dynamic microtubules were imaged using an Olympus BX51WI microscope equipped with × 20/0.5 N.A. and × 100/1.0 N.A. water-immersion dipping-cone objectives, an automated filter wheel (Sutter) and a cooled CCD camera (Retiga EXi; Qimaging), controlled by μManager [52] . Neutral density and infrared-blocking filters in the light path were used to prevent photo toxicity and photo bleaching. To follow EB3 comets, 200 images per movie were acquired at 0.5 Hz (2 Hz for analysis of comet track parameters) using an exposure time of 500 ms. For measuring paclitaxel effects, the drug was included in the superfusion solution (solvent, 0.2% dimethylsulphoxide) and comet densities were recorded repeatedly for up to 3 h. For analysis of degenerating and regenerating axons, mice were anesthetized with ketamine–xylazine (as above) and intercostal nerves were transected at the third rib [53] . After surgical closure of the wound, the mice were placed in a heated recovery chamber. Explants were prepared as described above after the desired interval. To image alterations in microtubule dynamics after acute axon cut, we performed laser axotomies in the triangularis sterni explant using an FV1000MPE two-photon microscope (Olympus). A femtosecond pulsed Ti:Sapphire laser (Mai Tai HP, Newport/Spectra Physics) tuned to 910 nm was placed on the axon for 3–5 s at 100% power using a × 100/1.0 N.A. water objective. The explants were then transferred to a wide-field setup and imaged as described above. To assay the effects of paclitaxel treatment on AAD, explants were pretreated for 1.5 h before laser axotomy. Time-lapse imaging in acute cerebellar slices To study microtubule dynamics in Purkinje cell dendrites, acute cerebellar slices of Thy1: EB3-YFP transgenic mice were prepared. Mice were lethally anesthetized with CO 2 and the cerebellum was rapidly removed and placed into oxygenated Ringer’s solution at 0–2 °C. Slices (300 μm thick) were cut using a vibratome slicer (Leica). After cutting, slices were kept at 34 °C for 1 h and then imaged for up to 4 h at 33–36 °C in oxygenated Ringer’s solution. Slices were imaged on an FV1000 confocal microscope (Olympus) using × 20/0.5 N.A. and × 100/1.0 N.A. water-immersion dipping-cone objectives. Imaging of microtubule dynamics in the spinal cord In vivo imaging of the lumbar spinal cord was carried out as previously described [54] , [55] . Briefly, mice were anaesthetized by an intraperitoneal injection of ketamine–xylazine (ketamine 87 mg kg −1 , xylazine 13 mg kg −1 ). Anesthesia was reapplied as needed (60–120 min). To access the dorsal surface of the lumbar spinal cord, a laminectomy was performed. To minimize movement during high-resolution imaging, the vertebral column was immobilized using compact spinal cord clamps (Narishige) [56] and mice were intubated following a tracheotomy. Symmetrical incisions were made lateral to the spinal column, one pair along the vertebral level rostral, and another pair two segments caudal to the laminectomy site for insertion of the spinal cord clamps. To allow for the formation of a liquid reservoir (regularly filled with prewarmed mouse artificial cerebrospinal fluid; aCSF: 148.2 NaCl, 3.0 KCl, 1.4 CaCl2, 0.8 MgCl2, 0.8 Na2HPO4, 0.2 NaH2PO4 in mM) and access with a water dipping-cone objective (× 25/1.05), an agarose well (2% agarose in aCSF) was made around the surgery site. Time-lapse recordings were acquired using an Olympus FVMPE-RS two-photon system equipped with a femtosecond pulsed Ti:Sapphire laser (Mai Tai HP, Newport/Spectra Physics). The laser was tuned to 930 nm for excitation of YFP. Detectors consisted of gallium arsenide phosphide photomultiplier tubes. All light was first filtered through a 690 nm short pass dichroic mirror. A 495–540 nm barrier filter in front of the gallium arsenide phosphide detectors was used for imaging YFP. Cranial window implantation and cortical in vivo imaging Cranial window implantation was performed as previously described [23] , [24] . In brief, mice were anesthetized with an intraperitoneal injection of ketamine–xylazine (ketamine 140 mg kg −1 , xylazine 10 mg kg −1 ). In addition, dexamethasone (6 mg kg −1 ) was injected intraperitoneally to prevent the development of cerebral oedema [24] . Mice were then placed on a heating blanket and stabilized in a stereotaxic frame. Using a dental drill (Schick-Technikmaster C1; Pluraden), a round craniotomy was made and immediately covered with round coverslip (3 mm). The coverslip was sealed to the skull using dental acrylic (Cyano-Veneer fast; Schein). A small metal bar was cemented next to the coverslip to allow repositioning of the mouse during subsequent imaging sessions. After surgery, mice received subcutaneous doses of the analgesic Carprofen (7.5 mg kg −1 ) and the antibiotic cefotaxime (5 mg kg −1 ). Imaging started 21 days after surgery to allow mice to recover and cranial windows to become clear. For time-lapse imaging of the somatosensory cortex, animals were anesthetized as described above and placed into a metal holder. Movies were acquired using the Olympus FVMPE-RS system as described for spinal cord imaging. Image analysis and processing To quantify comet parameters, images were analysed using the open-source software ImageJ/Fiji ( http://fiji.sc ) and the obtained movies were auto-aligned using the ‘ StackReg ’ algorithm [57] . Dynamic microtubules were analysed with the MTrackJ-plugin (developed by E. Meijering, Biomedical Imaging Group, Erasmus Medical Center, Rotterdam) by manual tracking of fluorescent EB3 comets that appeared on at least three consecutive frames. Polar plots were generated with IGOR software (WaveMetrics). Time-lapse movies recorded on scanning microscopes were de-noised using the CANDLE algorithm, a Matlab based software tool [58] . The following parameters were measured: orientation (angle of comet deviation measured from the local neurite orientation set to 0°), density of dynamic microtubules (average number of moving fluorescent comets in 200 frames in a random>50 μm 2 axon area expressed as comets μm −2 ) and average speed of EB3 comets (total displacement divided by observation time). For analysis of comet track parameters, movies at higher temporal resolution were obtained. ‘Pauses’ were identified as intervals during which the comet translocated less than 2 pixels (approximately the ‘jitter’ of our manual tracking; often the comet briefly dimmed or disappeared but resumed growth from the same position); ‘set-backs’ were phases, during which comets briefly disappeared and then reappeared further proximal along the same trajectory. A number of reasons prompted us to analyse comet density in two dimensions, although a full three-dimensional treatment seems more obvious at first glance. First, already when imaging in a single plane, recordings tend to be limited by temporal resolution and signal-to-noise constraints; three-dimensional analysis would result in severe under-sampling of comets with most microscope technologies. Furthermore, based on an estimate of the depth of field of our objectives, we believe that in most cases we capture comets in a subvolume of the relatively thick neurites that we imaged. Indeed, comet density did not correlate with neurite thickness or medial-to-lateral position within motor axons, as would be expected if a full cylinder was sampled (data not shown). As the depth of field can, however, not easily be measured, and in some thin neurites (for example, cortical dendrites) the above listed considerations argue that a certain volume error persists (which leads to an underestimate of volumetric comet density), we felt it to be more appropriate to restrict our analysis to area densities to be upfront about the limitations in the quantitative accuracy of our analysis. To quantify morphological features of neuromuscular junctions, confocal image stacks of fixed triangularis sterni explants from EB3-YFP-positive and -negative litter mates were analysed as follows. The size of neuromuscular junctions was determined by measurements of the thresholded area of Bungarotoxin staining on confocal stacks. The size of the muscle fibres was measured on rotated confocal projections as the circumference of individual fibres revealed by phalloidin staining. To measure the ratio of detyrosinated versus total tubulin, confocal images of antibody stainings were analysed in ImageJ/Fiji. A region of interest was placed within an axon of Thy1 :EB3-YFP transgenic mice and EB3-YFP-negative litter mates. Both channels were background subtracted and their ratio was determined in a single optical section. We determined the number of anterogradely and retrogradely transported mitochondria (‘transport flux’) in explants from MitoMice (line C) crossed to heterozygous Thy1 :EB3-YFP mice as the number of fluorescent mitochondria per minute that crossed a vertical line placed across the axon. For this purpose, time-lapse movies were obtained as described for imaging microtubule dynamics and results from transgenic and non-transgenic litter mates were compared. Electron micrographs were analysed using ImageJ/Fiji. Microtubule length and orientation were analysed on lateral sections of 25 μm axon segments where orientation angle of 0° was considered parallel to the axial direction of the axon. Microtubule density was analysed on cross-sections of random axons ranging between ~4–50 μm 2 . For image representation, confocal and wide-field images were combined after pseudocolouring using the ‘screen’ function in Photoshop and gamma was adjusted non-linearly in some images that illustrate qualitative properties to better reveal low-intensity objects. For overview images of expression patterns, multiple stitched frames were montaged in Photoshop. Montages of tiled confocal images are presented on a black background. Critical comparative data sets (for example, effects of paclitaxel on AAD and comet densities in SOD mice) were analysed by one or two blinded researchers. Statistics Sample sizes were determined on the basis of prior experience in previous experiments. Statistics were performed using Microsoft Excel and GraphPad PRISM software. Statistical significance was determined using two-tailed t -tests or analysis of variance where appropriate. P values<0.05 were considered to be significant and indicated by ‘*’; P values<0.01 were indicated by ‘**’ and<0.001 by ‘***’. Graphs show mean±s.e.m. Sample sizes in the text are given as n / m = n neurites from m mice, unless stated otherwise. How to cite this article : Kleele, T. et al . An assay to image neuronal microtubule dynamics in mice. Nat. Commun. 5:4827 doi: 10.1038/ncomms5827 (2014).